Editing the genome to introduce a beneficial naturally occurring mutation associated with increased fetal globin Genetic disorders resulting from defects in the adult globin genes are among the most common inherited diseases. Symptoms worsen from birth as fetal γ-globin expression is silenced. Genome editing could permit the introduction of beneficial single-nucleotide variants to ameliorate symptoms. Here, as proof of concept, we introduce the naturally occurring Hereditary Persistance of Fetal Haemoglobin (HPFH) −175T>C point mutation associated with elevated fetal γ-globin into erythroid cell lines. We show that this mutation increases fetal globin expression through de novo recruitment of the activator TAL1 to promote chromatin looping of distal enhancers to the modified γ-globin promoter. Normally, fetal haemoglobin (HbF) levels are downregulated postnatally to ∼ 1% of total haemoglobin; however, in some individuals, higher levels of HbF persist throughout adult life. This condition is known as Hereditary Persistence of Fetal Haemoglobin (HPFH) and has been shown to ameliorate the symptoms of both sickle-cell disease (SCD) and β-thalassaemia [1] . These diseases are typically managed by pharmacological agents such as hydroxyurea, which partially increase the production of HbF, blood transfusions or bone marrow transplants [2] . In the case of drug treatment, the level of efficacy is highly variable and not all patients respond satisfactorily [3] . Current research is thus focused on identifying modulators that can reactivate the expression of HbF in adult life [4] . The two human fetal globin genes G γ and A γ consist of highly similar stretches of DNA each spanning ∼ 5 kb ( Fig. 1a ). It is believed that they arose via a tandem duplication event [5] . The 5′ regulatory regions of the two γ -genes are identical up to position −221 upstream of the transcription start site. The rest of the 5-kb duplicated region differs on average in ∼ 14% of nucleotides [5] . During the fetal period, the G γ gene, which is closer to the powerful locus control region enhancer (LCR), is expressed about twice as strongly as the A γ gene [6] . 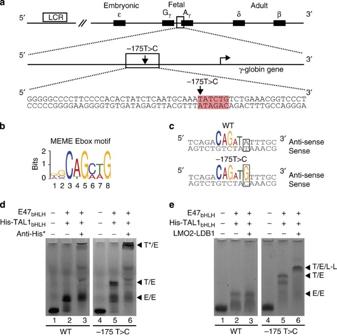Figure 1:The -175T>C mutation in theγ-globinpromoter creates an E-Box motif. (a) Schematic of the humanβ-globinlocus. Enlarged is theγ-globinproximal promoter. The position of the −175T>C mutation is indicated by a downward arrow. The newly created TAL1 consensus site is shown by a red box. (b) TAL1 consensus binding motif as determined by MEME analysis of published ChIP-seq data40. (c) The −175T>C mutation creates a complete E-Box consensus on the antisense strand of theγ-globinpromoter. Nucleotides at position −175 are shown in boxes. (d) EMSA. The DNA-binding domains (bHLH) of TAL1 and E47 were coexpressed in bacteria and purified by ion exchange chromatography. Binding of E47/E47 homodimer (E/E) and TAL1/E47 heterodimer (T/E) to the WT and −175T>Cγ-globinpromoters is shown in lanes 2 and 5, respectively. Lanes 1 and 4 show probe alone; specific binding of TAL1/E47 to the mutant probe is confirmed by supershift (T*/E) using an anti-His antibody (lane 6). The probe spans region −166 to −215. (e) EMSA showing interaction of TAL1/E47 with LMO2-LDB1 and the mutant −175T>C promoter. LMO2 and LDB1 were bacterially expressed as a tethered protein14and then purified by ion exchange chromatography. Binding of E47/E47 homodimer (E/E) and TAL1/E47 heterodimer (T/E) to the WT and −175T>Cγ-globinpromoters is shown in lanes 2 and 5, respectively. Lanes 1 and 4 show probe alone. The retarded band in lane 5 supershifts upon addition of LMO2-LDB1 (lane 6) indicating an interaction of TAL1/E47 with LMO2-LDB1 (T/E/L-L). The probe spans region −163 to −195. Figure 1: The -175T>C mutation in the γ-globin promoter creates an E-Box motif. ( a ) Schematic of the human β-globin locus. Enlarged is the γ-globin proximal promoter. The position of the −175T>C mutation is indicated by a downward arrow. The newly created TAL1 consensus site is shown by a red box. ( b ) TAL1 consensus binding motif as determined by MEME analysis of published ChIP-seq data [40] . ( c ) The −175T>C mutation creates a complete E-Box consensus on the antisense strand of the γ-globin promoter. Nucleotides at position −175 are shown in boxes. ( d ) EMSA. The DNA-binding domains (bHLH) of TAL1 and E47 were coexpressed in bacteria and purified by ion exchange chromatography. Binding of E47/E47 homodimer (E/E) and TAL1/E47 heterodimer (T/E) to the WT and −175T>C γ-globin promoters is shown in lanes 2 and 5, respectively. Lanes 1 and 4 show probe alone; specific binding of TAL1/E47 to the mutant probe is confirmed by supershift (T*/E) using an anti-His antibody (lane 6). The probe spans region −166 to −215. ( e ) EMSA showing interaction of TAL1/E47 with LMO2-LDB1 and the mutant −175T>C promoter. LMO2 and LDB1 were bacterially expressed as a tethered protein [14] and then purified by ion exchange chromatography. Binding of E47/E47 homodimer (E/E) and TAL1/E47 heterodimer (T/E) to the WT and −175T>C γ-globin promoters is shown in lanes 2 and 5, respectively. Lanes 1 and 4 show probe alone. The retarded band in lane 5 supershifts upon addition of LMO2-LDB1 (lane 6) indicating an interaction of TAL1/E47 with LMO2-LDB1 (T/E/L-L). The probe spans region −163 to −195. Full size image Genome editing has become an important technique to study human disease in in vivo models [7] and may one day become an established therapeutic approach to correct disease-causing mutations [8] . Here we have utilized transcription activator-like effector nuclease (TALEN)-mediated genome editing to introduce the naturally occurring −175T>C HPFH mutation into the γ-globin promoter in erythroid cell lines. We uncover the molecular mechanism behind the −175T>C HPFH mutation, demonstrating that it creates a de novo binding site for the erythroid transcriptional activator T-cell acute lymphocytic leukemia protein 1 (TAL1). We also show reactivation of fetal globin expression and enhanced looping of the LCR to the γ-globin promoter in these modified cell lines. The −175T>C HPFH mutation elevates HbF levels in humans At least eight individuals from five unrelated families (with different ethnic backgrounds) have been described who carry a T to C substitution at position −175 in the fetal γ-globin promoter ( Supplementary Table 1 ). Clinical data reveal that their HbF levels are strongly elevated and vary between 16 and 41% of total haemoglobin. Thus, this mutation is associated with HPFH in vivo [9] , [10] . A close inspection of this HPFH mutation revealed that the T>C substitution creates a consensus binding motif (E-Box) for the transcription factor TAL1 (best viewed on the antisense strand of the γ-globin promoter; Fig. 1a–c ). The −175T>C mutation creates a de novo TAL1-binding site TAL1 is a member of the basic helix–loop–helix (bHLH) family of transcription factors and is required for normal erythropoiesis [11] . It binds to DNA E-Box motifs of the sequence CANNTG and is often found as part of a multiprotein complex together with the LIM-only domain protein LMO2 and the LIM domain-binding protein LDB1, which in turn recruit other cofactors to regulate transcription [12] , [13] . To test the affinity of TAL1 for the mutated sequence, we expressed the DNA-binding domain of TAL1 and its cofactor E47, and compared binding with a wild-type (WT) and mutant (−175T>C) γ-globin promoter probe in electrophoretic mobility shift assays (EMSAs). A retarded protein–DNA complex corresponding to the TAL1/E47 heterodimer was observed only in the presence of the mutant probe, whereas we observed weak binding of the E47 homodimer to both probes ( Fig. 1d and Supplementary Fig. 1 ). In addition, we observed that upon addition of a tethered LMO2 and LDB1 (ref. 14 ) protein only the retarded TAL1/E47–DNA complex supershifted as LMO2 interacts with TAL1 but not E47 (refs 15 , 16 ; Fig. 1e ). TAL1 binds and activates γ-globin −175T>C in murine cells To confirm our findings in a cellular environment, we developed a strategy to introduce the −175T>C mutation into the genome of transgenic murine erythroleukaemia (MEL) cells. These cells carry a modified version of the human β-globin locus on a bacterial artificial chromosome (BAC) with dsRED and enhanced green fluorescent protein (EGFP) replacing the endogenous G γ and β-globin gene coding sequences, respectively ( Fig. 2a ) [17] . This fluorescent reporter system can be used to study mechanisms of globin switching as these cells express EGFP under the control of the adult human β-globin promoter, but retain the potential for reactivation of the silenced fetal γ-globin promoters [18] . To study the effect of the −175T>C mutation on γ-globin gene expression, we further modified this cell line using TALENs that target the A γ-globin gene promoter [19] . Using a homologous recombination strategy, we introduced the −175T>C substitution into the A γ promoter and incorporated an enhanced cyan fluorescent protein ( ECFP ) reporter gene ( Fig. 2a and Supplementary Fig. 2 ). As a control, we also generated clonal cell lines expressing ECFP under the control of the WT A γ promoter ( Fig. 2b ). Successful targeting was confirmed by genomic PCR with one primer located outside of the region contained in the targeting vector followed by sequencing of the promoter region ( Fig. 2c and Supplementary Fig. 3 ). 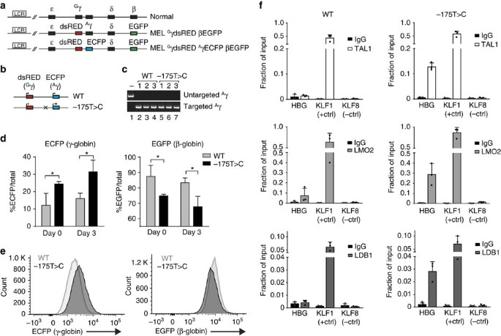Figure 2: The −175T>C mutation increases promoter activity in transgenic MEL cells. (a) Schematic of the unmodified humanβ-globinlocus (top), the locus in transgenic MEL cells before (middle) and after genome editing (bottom). (b) Schematic showing the modifiedγ-globingenes in MEL WT:Aγ or −175T>C:Aγ cells, respectively. (c) Genomic PCR using primers to distinguish between unmodified (upper panel) andAγ-globinpromoter-ECFP-targeted cells (lower panel). Lane 1 shows unmodified MEL cells; lanes 2–7 show genomic PCR for successfully modified clonal populations of MEL WT/−175T>C:Aγ cells. (d) Expression of reporter genes as determined by flow cytometry. Shown is the percentage of ECFP (Aγ-globin, left panel) and EGFP (β-globin, right panel) over total measurable globin reporters (ECFP, EGFP and dsRED) comparing clonal MEL WT:Aγ and −175T>C:Aγ cell populations (n=3) in uninduced state (day 0) and after 72 h of induction with 2% dimethylsulphoxide (day 3). ECFP expression is significantly upregulated in MEL −175T>C:Aγ cells, whereas EGFP expression is significantly downregulated. Significance was determined by unpaired two-tailedt-test (*P<0.05). Shown is mean±s.d. (e) Flow cytometry of clonal populations of MEL WT:Aγ or −175T>C:Aγ cells. Shown are superimposed representative histograms comparing expression levels of ECFP (Aγ-globin) and EGFP (β-globin) between 72 h-induced MEL WT:Aγ and −175T>C:Aγ cells. Depicted is the median of the monitored monoclonal populations (n=3) (f) anti-TAL1, anti-LMO2 and anti-LDB1 ChIP in MEL WT:Aγ (left panel) or −175T>C:Aγ (right panel) monoclonal cell populations (n=3). Significant enrichment of these factors is only seen at theγ-globinpromoter (HBG) carrying the −175T>C mutation (P<0.005 for TAL1,P<0.05 for LMO2 andP<0.01 for LDB1 as determined by unpaired two-tailedt-test). Shown is mean±s.d. Figure 2: The −175T>C mutation increases promoter activity in transgenic MEL cells. ( a ) Schematic of the unmodified human β-globin locus (top), the locus in transgenic MEL cells before (middle) and after genome editing (bottom). ( b ) Schematic showing the modified γ-globin genes in MEL WT: A γ or −175T>C: A γ cells, respectively. ( c ) Genomic PCR using primers to distinguish between unmodified (upper panel) and A γ-globin promoter- ECFP -targeted cells (lower panel). Lane 1 shows unmodified MEL cells; lanes 2–7 show genomic PCR for successfully modified clonal populations of MEL WT/−175T>C: A γ cells. ( d ) Expression of reporter genes as determined by flow cytometry. Shown is the percentage of ECFP ( A γ-globin, left panel) and EGFP (β-globin, right panel) over total measurable globin reporters (ECFP, EGFP and dsRED) comparing clonal MEL WT: A γ and −175T>C: A γ cell populations ( n =3) in uninduced state (day 0) and after 72 h of induction with 2% dimethylsulphoxide (day 3). ECFP expression is significantly upregulated in MEL −175T>C: A γ cells, whereas EGFP expression is significantly downregulated. Significance was determined by unpaired two-tailed t -test (* P <0.05). Shown is mean±s.d. ( e ) Flow cytometry of clonal populations of MEL WT: A γ or −175T>C: A γ cells. Shown are superimposed representative histograms comparing expression levels of ECFP ( A γ-globin) and EGFP (β-globin) between 72 h-induced MEL WT: A γ and −175T>C: A γ cells. Depicted is the median of the monitored monoclonal populations ( n =3) ( f ) anti-TAL1, anti-LMO2 and anti-LDB1 ChIP in MEL WT: A γ (left panel) or −175T>C: A γ (right panel) monoclonal cell populations ( n =3). Significant enrichment of these factors is only seen at the γ-globin promoter (HBG) carrying the −175T>C mutation ( P <0.005 for TAL1, P <0.05 for LMO2 and P <0.01 for LDB1 as determined by unpaired two-tailed t -test). Shown is mean±s.d. Full size image We then investigated expression levels of ECFP ( A γ-globin) and EGFP (β-globin) by flow cytometry. ECFP ( A γ) expression was significantly higher in −175T>C cells compared with WT, whereas expression of EGFP (β-globin) was lower in those cells ( Fig. 2d,e ). The differences increased further upon differentiation of the cells for 3 days. In contrast to the A γ-globin gene that was modified, the unmodified G γ-globin locus, marked by the expression of dsRED driven by the WT G γ , remained unchanged ( Supplementary Fig. 4a ). We also investigated whether the −175T>C mutation facilitates in vivo binding of TAL1 to the γ-globin promoter in the cell lines. Chromatin immunoprecipitation (ChIP) experiments revealed a significant enrichment of TAL1 occupancy at the γ -promoter in the presence of the −175T>C mutation ( Fig. 2f ). We then assayed for occupancy of the TAL1 partner proteins LMO2 and LDB1 at the mutated promoter. Both LMO2 and LDB1 ChIP revealed enrichment of these factors at the γ-globin promoter in cells carrying the −175T>C mutation ( Fig. 2f ). In addition, we performed ChIP experiments for GATA1, an erythroid transcription factor previously demonstrated to bind the −175 region in vitro [9] , [20] , in both MEL: A γ WT and −175T>C: A γ cells. There was a modest 1.7-fold increase in GATA1 binding to the γ-globin promoter when the mutation was present but this increase was not statistically significant ( P =0.19 as determined by unpaired two-tailed t -test; Supplementary Fig. 4b ). TAL1 binds and activates γ-globin −175T>C in human cells We next used the same TALEN-based approach in human erythroid K562 cells. Our strategy here was to place a fluorescent tdTomato reporter under the control of either a WT or −175T>C G γ-globin promoter. The TALEN targeting is such that it cuts both γ-globin genes and accordingly the recombination generates a single fetal globin gene driven either by a WT promoter or the −175T>C promoter depending on the donor vector supplied ( Fig. 3a and Supplementary Fig. 2 ). Hence, the tdTomato reporter represents total expression of the fetal globin genes. We established clonal K562 cell lines, which will be referred to as K562 WT/− 175T>C: G γ - A γ. 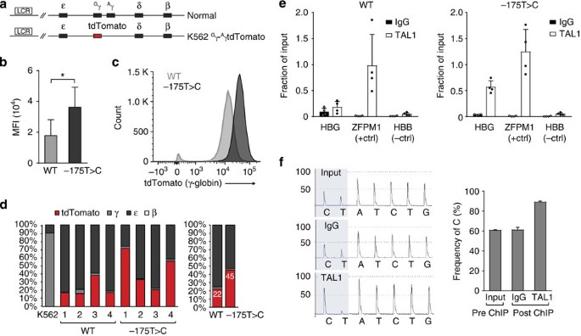Figure 3: The −175T>C HPFH mutation increases promoter activity in K562 cells. (a) Schematic of the normal (top) and engineered (bottom)β-globinlocus in K562 cells. (b) Bar chart showing mean±s.d.γ-globin(tdTomato) promoter activity for clonal populations (n=5) of K562 WT/-175T>C:Gγ-Aγcells as determined by measuring median tdTomato fluorescence intensity. Significance was determined by unpaired two-tailedt-test (*P<0.05). (c) Histogram showingγ-globinpromoter activity in representative clonal populations of K562 WT/−175T>C:Gγ-Aγcells, as determined by tdTomato fluorescence. Depicted is the median out of five clonal populations (for K562 WTGγ-Aγor −175T>C:Gγ-Aγ, respectively). (d) Shown is the percentage mRNA expression ofβ-like globinsin unmodified K562 cells (left) and also expression oftdTomatoandβ-like globinsin clonal populations of K562 WT/−175T>C:Gγ-Aγcells as determined by qPCR. The graph on the right depicts mean mRNA levels for clonal K562 WT/−175T>C:Gγ-Aγcell populations (n=4). (e) Anti-TAL1 ChIP in K562 WT/-175T>C:Gγ-Aγcells lines (n=4). Shown is mean±s.d. Enrichment of TAL1 atγ-globinpromoter (HBG) is significantly higher in K562 −175T>C:Gγ-Aγcells (P<0.005). Significance was determined by unpaired two-tailedt-test. (f) Representative sequencing pyrograms (left) of PCR products derived from input and ChIP samples in K562 cells heterozygous for the −175T>C mutation. Shown on the right is the mean frequency of cytosine (=mutated allele) at position −175 of theγ-globinpromoter in input, control antibody ChIP (IgG) and TAL1 ChIP. The mutated allele is enriched only after TAL1 ChIP. Pyrosequencing was performed in triplicate and shown is the mean±s.d. Figure 3: The −175T>C HPFH mutation increases promoter activity in K562 cells. ( a ) Schematic of the normal (top) and engineered (bottom) β-globin locus in K562 cells. ( b ) Bar chart showing mean±s.d. γ-globin ( tdTomato ) promoter activity for clonal populations ( n =5) of K562 WT/-175T>C: G γ - A γ cells as determined by measuring median tdTomato fluorescence intensity. Significance was determined by unpaired two-tailed t -test (* P <0.05). ( c ) Histogram showing γ-globin promoter activity in representative clonal populations of K562 WT/−175T>C: G γ - A γ cells, as determined by tdTomato fluorescence. Depicted is the median out of five clonal populations (for K562 WT G γ - A γ or −175T>C: G γ - A γ , respectively). ( d ) Shown is the percentage mRNA expression of β-like globins in unmodified K562 cells (left) and also expression of tdTomato and β-like globins in clonal populations of K562 WT/−175T>C: G γ - A γ cells as determined by qPCR. The graph on the right depicts mean mRNA levels for clonal K562 WT/−175T>C: G γ - A γ cell populations ( n =4). ( e ) Anti-TAL1 ChIP in K562 WT/-175T>C: G γ - A γ cells lines ( n =4). Shown is mean±s.d. Enrichment of TAL1 at γ-globin promoter (HBG) is significantly higher in K562 −175T>C: G γ - A γ cells ( P <0.005). Significance was determined by unpaired two-tailed t -test. ( f ) Representative sequencing pyrograms (left) of PCR products derived from input and ChIP samples in K562 cells heterozygous for the −175T>C mutation. Shown on the right is the mean frequency of cytosine (=mutated allele) at position −175 of the γ-globin promoter in input, control antibody ChIP (IgG) and TAL1 ChIP. The mutated allele is enriched only after TAL1 ChIP. Pyrosequencing was performed in triplicate and shown is the mean±s.d. Full size image K562 cell lines are often aneuploid [21] , [22] , and karyotyping of chromosome 11 revealed our lines to be triploid for the β-globin locus ( Supplementary Fig. 5a ). We therefore selected clones where successful homologous recombination had introduced tdTomato into all three endogenous γ-globin loci and chose recombinant cell lines that carried the WT promoter or −175T>C substitution driving tdTomato at one or more of these three alleles ( Supplementary Fig. 3 ). To analyse the effect of introducing the −175T>C mutation, we performed flow cytometry on the K562 WT/ − 175T>C: G γ - A γ cell lines and determined the expression levels of tdTomato ( Fig. 3b,c ). On average, clones carrying the −175T>C mutation in at least one allele showed a twofold higher median fluorescence than clones with tdTomato under the control of the WT γ-globin promoter. We also determined the percentage mRNA expression for each of the β-like globin genes and found again that −175T>C mutant clones on average showed a twofold higher tdTomato mRNA expression than K562 WT: G γ - A γ cells ( Fig. 3d ). To confirm that differences in γ-globin expression were not associated with altered expression of other transcription factors involved in erythroid gene regulation, we analysed expression of TAL1, GATA1 and GATA2 (refs 23 , 24 ) and two well-known silencers of fetal globin expression, SOX6 and BCL11A (refs 25 , 26 ; Supplementary Fig. 5b ). We compared clonal populations of K562 WT and − 175T>C: G γ - A γ cells, along with unmodified K562 cells, and found no significant differences in transcription factor expression between samples. We then performed TAL1 ChIPs in clonal K562 WT and − 175T>C: G γ - A γ cell lines ( Fig. 3e ). We found that TAL1 binds to the γ-globin promoter in K562 − 175T>C: G γ - A γ but not WT cells. Preferential binding of TAL1 to the −175T>C γ-globin promoter was also confirmed by pyrosequencing of input and ChIP PCR products from K562 clones heterozygous for the mutation ( Fig. 3f ). Before immunoprecipitation, the allelic constitution of the promoter is heterozygous with ∼ 40% T (WT) and ∼ 60%°C (mutation). ChIP with TAL1 antibody showed enrichment for the mutant allele (90%), whereas control IgG antibody precipitated the input ratio of 40:60 WT:mutant allele, strongly supporting the hypothesis that the −175T>C mutation directly creates a novel TAL1-binding site. −175T>C increases enhancer looping to the γ-globin promoter Developmental regulation of the β-globin locus is controlled by progressive looping of distal enhancer elements in the locus control region to the promoters of the embryonic, fetal and adult β-like globin genes [24] . Recently, it has been shown that that an artificial zinc-finger protein tethered to the self-association domain of LDB1 can force looping of the γ-globin promoter to override this developmentally regulated gene expression programme [27] , [28] . Our hypothesis is that the −175T>C substitution similarly creates a new TAL1/LDB1-binding site, and thus may also promote looping of the LCR to the γ-globin promoter. To test this hypothesis, we performed chromatin conformation capture (3C) experiments in the transgenic MEL cell lines and the modified K562 cells ( Fig. 4 and Supplementary Fig. 6 ). Relative crosslinking frequencies between hypersensitive site 2 and the A γ promoter were consistently higher in MEL cells carrying the −175T>C mutation compared with WT controls. In K562 cells, we saw an increase in crosslinking frequencies between the γ-globin promoter and all hypersensitive sites in −175T>C-modified cells compared with cells incorporating the WT promoter tdTomato construct. Thus, we suggest that the −175T>C mutation enhances chromatin looping to the A γ promoter to activate expression of fetal globins. 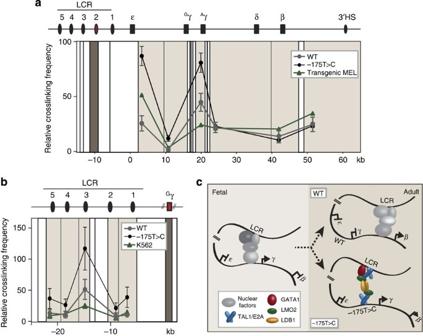Figure 4:Chromatin looping of the locus control region to theγ-globinpromoter. (a) 3C assay measuring locus-wide crosslinking frequencies in MEL WT:Aγ cells (grey), MEL −175T>C:Aγ cells (black) and unmodified transgenic MEL cells (green). A schematic of the humanβ-globinlocus is shown on top of the graph. Thexaxis indicates distances in kb from theɛ-gene. Vertical lines represent HindIII restriction sites. The dark brown bar denotes the anchor HindIII fragment containing hypersensitive site (HS) 2. Beige bars denote analysed HindIII fragments. Replicates are from two independently generated clonal cell populations for WT:Aγ and −175T>C:Aγ cells (n=2), respectively. Shown is mean±s.e.m. (b) 3C assay measuring relative crosslinking frequencies ofGγ-globin and LCR in K562 WT and −175T>C:Gγ-Aγcells. Vertical lines represent HindIII restriction sites. The dark brown bar denotes the anchor HindIII fragment containing theGγ-globinpromoter. Replicates are from independently generated clonal cell populations of K562 WT (n=2) and −175T>C:Gγ-Aγ(n=3). Shown is mean±s.e.m. (c) Model of LCR looping to theγ-globinpromoter upon introduction of the −175T>C mutation in theγ-globinpromoter. In the fetal environment, nuclear factors mediate looping of the LCR to theγ-globingenes (left panel). In the WT adult environment, the LCR loops to theβ-globingene andγ-globinis silenced. The −175T>C mutation drives recruitment of the LCR to theγ-promoter via assembly of a looping complex consisting of TAL1 and associated cofactors41. Figure 4: Chromatin looping of the locus control region to the γ-globin promoter. ( a ) 3C assay measuring locus-wide crosslinking frequencies in MEL WT: A γ cells (grey), MEL −175T>C: A γ cells (black) and unmodified transgenic MEL cells (green). A schematic of the human β-globin locus is shown on top of the graph. The x axis indicates distances in kb from the ɛ-gene . Vertical lines represent HindIII restriction sites. The dark brown bar denotes the anchor HindIII fragment containing hypersensitive site (HS) 2. Beige bars denote analysed HindIII fragments. Replicates are from two independently generated clonal cell populations for WT: A γ and −175T>C: A γ cells ( n =2), respectively. Shown is mean±s.e.m. ( b ) 3C assay measuring relative crosslinking frequencies of G γ-globin and LCR in K562 WT and −175T>C: G γ - A γ cells. Vertical lines represent HindIII restriction sites. The dark brown bar denotes the anchor HindIII fragment containing the G γ-globin promoter. Replicates are from independently generated clonal cell populations of K562 WT ( n =2) and −175T>C: G γ - A γ ( n =3). Shown is mean±s.e.m. ( c ) Model of LCR looping to the γ-globin promoter upon introduction of the −175T>C mutation in the γ-globin promoter. In the fetal environment, nuclear factors mediate looping of the LCR to the γ-globin genes (left panel). In the WT adult environment, the LCR loops to the β-globin gene and γ-globin is silenced. The −175T>C mutation drives recruitment of the LCR to the γ -promoter via assembly of a looping complex consisting of TAL1 and associated cofactors [41] . Full size image Reactivating the expression of HbF in adult life has been a major therapeutic target of haemoglobinopathy research for decades and a number of different approaches to reactivation have been taken. We believe one elegant approach may be to introduce naturally occurring HPFH mutations to drive high HbF levels in adult red blood cells as these mutations are known to naturally ameliorate the symptoms of SCD and β-thalassaemia [16] . This approach has significant advantages as only naturally occurring variants are introduced and problems with epigenetic silencing of foreign genetic material or the unintended activation of nearby genes should be avoided. Here, we successfully edited the genome of erythroid cell lines to introduce the −175T>C HPFH mutation, and found that this was associated with a significant increase in γ-globin promoter activity. We therefore propose that this study presents a proof-of-concept model of a novel gene therapeutic strategy to reactivate the expression of γ-globin in adulthood. Nevertheless, further work will be required to overcome challenges in obtaining high-frequency recombination in pluripotent cells, obtaining enough cells for transplant, and assessing the safety of potential off-target effects. Most importantly, our models enabled us to determine the molecular mechanism that allows this HPFH mutation to facilitate persistent γ-globin expression. We showed that the −175T>C mutation creates a novel binding site for the activator TAL1. Indeed, our data indicate that TAL1 binds to the mutant γ-globin promoter in a complex with LMO2 and LDB1. It has recently been shown that LDB1 is the key factor enabling LCR looping to the globin genes, and that an artificial zinc-finger LDB1 construct is sufficient to force LCR looping to either the fetal or adult globin genes [28] . Our data suggest that recruitment of LDB1 to the γ-globin promoter by de novo binding of TAL1 can also facilitate looping to the LCR via dimer or multimerization [29] with LDB1 proteins ( Fig. 4c ). GATA1 has also been shown to work in combination with TAL1 to activate erythroid genes [30] , [31] , [32] , and interestingly there is an existing GATA1 consensus binding site near to the newly formed TAL1 site. From our data it is not clear if altered GATA1 binding also plays a critical role in activating γ-globin expression in the −175T>C HPFH model. We could show in vitro that mutual binding of TAL1 and GATA1 to the γ-globin promoter is possible when a bridging molecule LMO2/LDB1 is present ( Supplementary Fig. 1b,c ). Yet in ChIP experiments, we were unable to observe significant differences in GATA1 binding to the WT and −175T>C sequences. We have not examined the role of OCT1/POU2F1, which has also been reported to bind to this region of the γ-globin promoter in vitro [20] , [33] , [34] . Together, our findings provide a mechanistic explanation for how the −175T>C mutation results in HPFH and suggest a new approach in reactivating γ-globin expression in adult cells. By reversing globin switching, the engineering of this HPFH mutation increases expression of beneficial γ-globin and also reduces levels of defective β-globin chains, making this a possible future therapy for haemoglobinopathies such as SCD. Electrophoretic mobility shift assays DNA-binding assays were performed using 5′ fluorescein-labelled double-stranded DNA probes (Sigma-Aldrich). WT −166 to −215: 5′-Flc- TCCTCTTGGGGGCCCCTTCC CCACACTATCTCAATGCAAATATCTGTCTG -3′ Mutant −166 to −215: 5′-Flc- TCCTCTTGGGGGCCCCTTCC CCACACTATCTCAATGCAAACATCTGTCTG -3′ WT −163 to −195: 5′-Flc- CCCCACACTATCTCAATGCAAATATCTGTCTGAAA -3′ Mutant −163 to −195: 5′-Flc- CCCCACACTATCTCAATGCAAACATCTGTCTGAAA -3′ Probes for Supplementary Fig. 1a,b were radiolabelled with 32 P. WT −151 to −186: 5′- CTCAATGCAAATATCTGTCTGAAACGGTCCCTGGC -3′ Mutant −151 to −186: 5′- CTCAATGCAAACATCTGTCTGAAACGGTCCCTGGC -3′ WT −151 to −203: 5′- CCCCACACTATCTCAATGCAAATATCTGTCTGAAACGGTCCCTGGC -3′ Mutant −151 to −203: 5′- CCCCACACTATCTCAATGCAAACATCTGTCTGAAACGGTCCCTGGC -3′ Bacterial protein expression and purification were conducted as follows as previously described. GATA1 ZF was overexpressed in Escherichia coli BL21 (DE3). LMO2-LDB1 was expressed as a tethered protein [14] . Proteins were purified using a cation exchange column. TAL1 bHLH and E47 bHLH were coexpressed in the same host. Bacterial lysates of TAL1/E47 were first purified by cation exchange and then further purified with a nickel-nitrilotriacetic acid (Ni-NTA) affinity resin, and bound heterodimers were eluted with imidazole. Before EMSA, proteins were dialysed in dialysis buffer (150 mM NaCl, 10 mM Tris-HCl and 1 mM dithiothreitol, pH 8.0). They were then incubated with labelled oligo (5 nM) in mobility shift buffer (MSB) buffer (10 mM HEPES, pH 7.9, 30 mM NaCl and 1 mM MgCl 2 ) for 30 min at 4 °C. Ficoll loading dye was added to the reaction and samples were loaded onto an 8% non-denaturing polyacrylamide gel in 0.5 × Tris–borate–EDTA and subjected to electrophoresis at 17 mA for 2 h at room temperature (RT). After electrophoresis, gels were imaged using a Typhoon FLA-9500 imager (GE Healthcare Life Sciences). Nuclear extracts for EMSA were obtained from induced (72 h with 2% dimethylsulphoxide) MEL cells. An amount of 20 μg of total protein was used for each shift. Extracts were incubated with labelled oligos as described above. Cell lines and nucleofection K562 cells were maintained in RPMI1640 (Life Technologies) supplemented with 10% fetal calf serum (FCS; Life Technologies) and 1 × penicillin, streptomycin and L -glutamine (Life Technologies). The mouse erythroleukaemia (MEL) cells used for nucleofections carry the human β-globin locus on a 188-kb BAC with dsRED as a reporter under the control of G γ-globin promoter and EGFP under the control of the β-globin promoter [17] . These MEL G γdsREDβEGFP cells were maintained in the same media as K562 cells. Cells were transfected by nucleofection using a Neon Transfection System (Life Technologies). Cells (10 5 ) were resuspended in nucleofection buffer T (Neon Transfection Kit, Life Technologies) and given three pulses of 1,450 V for 20 ms. Cells were then cultured for 48–72 h in RPMI1640 supplemented with 10% FCS before selection. Tal-Effector-Nucleases and targeting vector construction γ-globin TALENs and targeting vector (tdTomato) were kindly donated by Matthew H. Porteus (Stanford University, CA) [19] . TALENs are described in Voit et al . [19] . They are expressed from a pcDNA3.1 (Invitrogen) vector driven by a cytomegalovirus (CMV) promoter. They were synthesized using a Golden Gate cloning strategy [35] with a Δ152 N-terminal domain and a +63 C-terminal domain [36] . The −175T>C mutation was introduced into the targeting vector by site-directed mutagenesis (Q5 SDM Kit, New England Biolabs), and its presence was confirmed by Sanger sequencing (Australian Genome Research Facility). A targeting vector containing ECFP in place of tdTomato was generated by PCR from pECFP-C1 (Clontech) for the ECFP fragment (F: 5′- CTCCTAGTCCAGACGCCATGGTGAGCAAGGGCGAG -3′, R: 5′- ATTAATGCATTTACTTGTACAGCTCGTCCATGCC -3′) and PCR from tdTomato targeting vector for the 5′ γ-promoter region (F: 5′- ATTAAAGCTTGATATCGAATTCGATT -3′, R: 5′- GGCGTCTGGACTAGGAG -3′) followed by overlap extension PCR of both fragments (F: 5′- ATTAAAGCTTGATATCGAATTCGATT -3′, R: 5′- ATTAATGCATTTACTTGTACAGCTCGT -3′). The resulting PCR product 5′γ-ECFP was then ligated into the target vector backbone via the restriction enzyme sites HindIII and NsiI. Generation of fluorescent reporter cell lines MEL G γdsREDβEGFP cells (10 5 ) were nucleofected with 2.5 μg of targeting vector (ECFP) and 500 ng of each TALEN plasmid ( Supplementary Fig. 2 ). Positively targeted cells were enriched by treatment with 1 mg ml −1 G418 (Geneticin, Life Technologies) for 5 days. Cells were then sorted for live cells with a BD Influx Cell Sorter (BD Biosciences, Cytopeia, USA) using the cell sorting service of the BRIL Flow Cytometry Facility (Mark Wainwright Analytical Centre, UNSW) to obtain single-cell clones. Targeting was then confirmed by genomic PCR spanning the integration junctions F: 5′- agtgtgtggactattagtcaa -3′, R: 5′- ATGAACTTCAGGGTCAGCTT -3′ and Sanger sequencing of PCR products. Engineered clonal populations were maintained in RPMI1640 (Life Technologies) supplemented with 10% FCS (Life Technologies) and 1 × penicillin, streptomycin and L -glutamine (Life Technologies). Differentiation of MEL cells was induced by adding 2% dimethylsulphoxide to the culture medium for a minimum of 3 and up to 10 days. K562 cells (10 5 ) were nucleofected in a similar way but with a targeting vector containing tdTomato as a fluorescent reporter. Targeted cells were enriched by treatment with 500 μg ml −1 G418 for 3 days and then sorted with a BD Influx Cell Sorter (BD Biosciences) for tdTomato -positive cells to establish single-cell clones. Targeting was confirmed by genomic PCR, F: 5′- agtgtgtggactattagtcaa -3′, R: 5′- atgaactctttgatgacctcc -3′. Genotypes were determined by genomic PCR using three primers, F: 5′- agtgtgtggactattagtcaa -3′, R1: 5′- atgaactctttgatgacctcc -3′ and R2: 5′- CAGTGGTATCTGGAGGACA -3′. Primer F and R1 amplify DNA from the modified γ-globin locus ( tdTomato positive, ∼ 1,200 bp), whereas Primer F and R2 amplify DNA from the unmodified γ-globin locus ( ∼ 2,500 bp). Only clones that were modified with tdTomato in all three alleles were selected for further studies. Homologous recombination did not always result in the introduction of the −175T>C mutation in all three alleles of chromosome 11, hence clones that had one or more alleles carrying the mutation were chosen for further studies. Clonal populations were then cultured in the same media as the engineered MEL cells. Analysis of mRNA expression mRNA from modified K562 G γ - A γ tdTomato cells was harvested by TRIReagent/chloroform (Sigma-Aldrich) extraction and purified on RNeasy columns (Qiagen). 5–10 μg of total RNA was used to synthesize cDNA with the SuperScript VILO cDNA Synthesis Kit (Life Technologies). Samples were assayed by quantitative real time PCR (qRT–PCR) with a FLEXSix Fluidigm Dynamic Array integrated fluidic circuit (Fluidigm) using EvaGreen dye on a BioMark System (Fluidigm). Primer sequences can be found in Supplementary Table 1 . Analysis of ECFP and EGFP expression ECFP, EGFP and dsRED expression of successfully modified MEL cell G γdsRED A γECFPβEGFP clones was monitored by flow cytometry using a BD LSRFortessa flow cytometer (BD Biosciences). Data were analysed using FACSDiva (BD) and FlowJo (Tree Star Inc.) software. Chromatin immunoprecipitation ChIP was performed using ∼ 5 × 10 7 cells per experiment [37] . Cells were crosslinked with 1% formaldehyde (Sigma-Aldrich) for 10 min at RT and reaction was quenched with glycine at a final concentration of 125 mM. For LDB1 ChIP, cells were crosslinked with ethylene glycol bis(succinimidyl succinate) (EGS) at a final concentration of 1.5 mM for 30 min followed by 1% formaldehyde crosslinking for 10 min. Crosslinked cells were then lysed and sonicated to obtain ∼ 200–300 bp fragments of chromatin. DNA was pulled down at 4 °C overnight using antibodies (15 μg) specific for TAL1/SCL (sc-12984 X, Santa Cruz Biotechnology), LMO2 (AF2726, R&D Systems), LDB1 (sc-11198 X, Santa Cruz Biotechnology), GATA1 (sc-265 X, Santa Cruz Biotechnology) or a negative control goat IgG (sc-2028, Santa Cruz Biotechnology). Chromatin was then reverse crosslinked and eluted at 65 °C overnight and DNA was purified. Real-time qPCR was performed on ChIP material using the primers in Supplementary Table 2 on a 7500 Fast Real-Time PCR System (Applied Biosystems). Relative alleleic quantification of immunoprecipitated DNA Quantity of WT or −175T>C alleles before and after ChIP was determined by pyrosequencing. ChIP material was amplified with primers F: 5′-biotin- CAAGGCTATTGGTCAAGGCAA -3′ and R: 5′- TTCCCCACACTATCTCAATGCAAA -3′ on a 7500 Fast Real-Time PCR System (Applied Biosystems). Pyrosequencing was performed using AGRF’s PyroMark Sequencing Service (Qiagen) with sequencing primer 5′- CACACTATCTCAATGCAAA -3′. Chromatin conformation capture The 3C assay was performed using ∼ 5 × 10 6 cells per experiment. Cells were crosslinked with 1.5% formaldehyde at room temperature for 10 min, followed by glycine quenching, cell lysis, HindIII (1,000 U) digestion overnight and T4 ligation (400 U) for 4–5 h at 16 °C followed by 30 min at room temperature (both New England Biolabs). 3C ligation products were quantified in triplicates by real-time qPCR. Primer sequences were previously described [38] and are listed in the Supplementary Table 2 . Primers were tested by serial dilution and gel electrophoresis to ensure specific and linear amplification ( Supplementary Fig. 6c,d ). Digestion efficiencies were monitored by qPCR with primer pairs that amplify genomic regions spanning or avoiding HindIII digestion sites ( Supplementary Fig. 6b ). Only samples with efficiencies >75% were considered for analysis. A BAC containing the entire human β-globin locus (pEBAC G γdsREDβEGFP) [39] was digested with HindIII and religated to generate random ligation products of HindIII fragments for transgenic MEL cell experiments ( Supplementary Fig. 6a ). For the 3C in K562s, we used a BAC containing the unmodified human β-globin locus (pBAC 148β). The ligated BAC DNA was serially diluted and used to generate standard curves for each primer pair to which all 3C products were normalized. The 3C signals at the β-globin locus were further normalized to those from an intervening genomic region. Statistical analysis Statistical analysis was performed using GraphPad Prism software. Significance was determined by unpaired two-tailed t -test using the Holm–Sidak method. How to cite this article: Wienert, B. et al . Editing the genome to introduce a beneficial naturally occurring mutation associated with increased fetal globin. Nat. Commun. 6:7085 doi: 10.1038/ncomms8085 (2015).